Failure to apply standard limit-of-detection or limit-of-quantitation criteria to specialized pro-resolving mediator analysis incorrectly characterizes their presence in biological samples 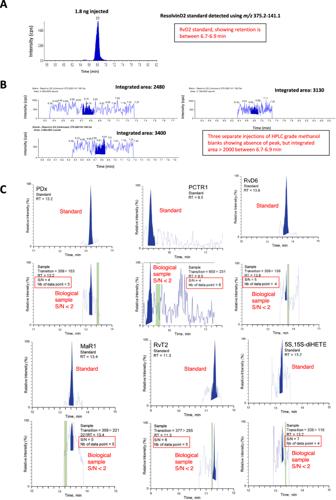Fig. 1: Analysis of methanol blanks shows integrated peak areas >2000 cps for RvD2, while flawed S/N analysis shows false positives for several SPM in Gomez et al. AExample chromatogram from 1.8 ng RvD2 standard analyzed using LC-MS/MS as described in Methods.BThree separate analyses of a methanol injection, in the region where RvD2 elutes showing the areas where the signal was integrated.CChromatograms taken directly from the Supplementary information of Gomez et al1. The chromatograms are representative of many from Supplementary information, in Gomez et al1, showing the authentic standard on top with analysis of the biological sample immediately below. In BLUE are the peaks areas computed by Gomez et al1and the green strips are the regions the authors used to calculate S/N ratios of 4, 4, 5, 7, 6 and 5, reading clockwise from the top left panel. In Red, we have added to the originals for clarification: labels of Standard, Biological Sample, a box around the original S/N, and estimations of S/N < 2, considering the SPM signal and the entire available baseline. 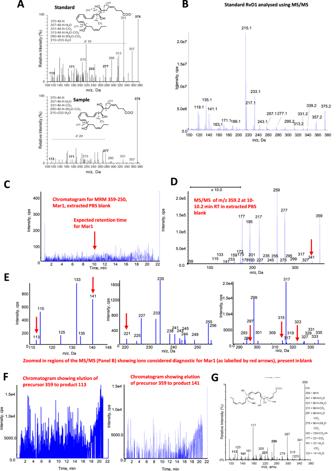Fig. 2: MS/MS of RvD1 do not match between standard and sample, and an extracted buffer blank shows absence of peak, but several detectable “diagnostic” ions for Mar1, with some being detected throughout the entire run. AScreenshot of Supplementary Fig.1Ashowing MS/MS of standard and sample, from Gomez et al.BMS/MS of an RvD1 standard generated in one of our laboratories.CChromatogram, monitoring for Mar1 atm/z359–250.DMS/MS at 10–10.2 min, where the Mar1 standard elutes, showing isolation and fragmentation of ion atm/z359.EZoomed in regions of centroid spectrum showing background ions contain several “diagnostic” ions for Mar1, as labelled by red arrows.FIons atm/z113 or 141 that are detected following fragmentation of m/z 359 are detected throughout the chromatographic run. Panel G. Figure showing first report of Mar1 MS/MS spectrum from12.GReproduced from Serhan et al.12, the first report of maresin-1 (Mar1) as a novel metabolite of DHA. See Supplementary Methods. Reporting summary Further information on research design is available in the Nature Portfolio Reporting Summary linked to this article.